Inhibition of PDE4B suppresses inflammation by increasing expression of the deubiquitinase CYLD The deubiquitinase CYLD acts as a key negative regulator to tightly control overactive inflammation. Most anti-inflammatory strategies have focused on directly targeting the positive regulator, which often results in significant side effects such as suppression of the host defence response. Here, we show that inhibition of phosphodiesterase 4B (PDE4B) markedly enhances upregulation of CYLD expression in response to bacteria, thereby suggesting that PDE4B acts as a negative regulator for CYLD. Interestingly, in Cyld-deficient mice, inhibition of PDE4B no longer suppresses inflammation. Moreover, PDE4B negatively regulates CYLD via specific activation of JNK2 but not JNK1. Importantly, ototopical post-inoculation administration of a PDE4 inhibitor suppresses inflammation in this animal model, thus demonstrating the therapeutic potential of targeting PDE4. These studies provide insights into how inflammation is tightly regulated via the inhibition of its negative regulator and may also lead to the development of new anti-inflammatory therapeutics that upregulate CYLD expression. Inflammation is a hallmark of many important human diseases including infectious diseases, chronic obstructive pulmonary diseases (COPD), otitis media (OM), asthma, arthritis, inflammatory bowel disease, atherosclerosis and cancer [1] , [2] , [3] , [4] . Although an appropriate inflammatory response is essential for eradicating pathogens, when excessive, it is clearly detrimental to the host [5] . Thus, inflammation must be tightly regulated [4] , [6] . However, how this response is controlled in inflammatory diseases remains largely unknown. Moreover, despite the enormous efforts that have been put into developing anti-inflammatory agents, to date, there has been limited success in developing therapies for long-term treatment of inflammatory disorders without significant side effects. Over the past decades, most strategies have focused on directly targeting the positive pathways, for example, the IκB kinase β (IKKβ), to suppress inflammation [7] . Although these agents often showed reasonable efficacy, they exhibited significant adverse effects, for example, increased susceptibility to infection and induction of apoptosis, which prevented their further clinical use [8] , [9] . Thus, there is an urgent need for developing novel therapeutic strategies without causing serious side effects by avoiding the direct targeting of the positive regulators of inflammation. In comparison with the positive regulators of inflammation, for example, IKKβ, the negative regulators, in particular inducible negative feedback regulators, have been shown to have a critical role in its tight control, thus preventing overactive and detrimental inflammatory responses. Recent studies have identified cylindromatosis (CYLD) as a key inducible negative feedback regulator of bacteria-induced inflammation [10] , [11] . CYLD is a novel deubiquitinase and has been shown to act as a negative regulator for various signalling pathways, for example, TRAF6, NEMO and Akt by removing lysine 63-linked polyubiquitin chains from several specific substrates [12] , [13] . Mutations of CYLD can lead to the development of tumours [14] , [15] . In addition to mutations, dysregulated expression of CYLD has also been reported under various pathological conditions. For instance, the expression of CYLD is relatively low under physiological conditions but is significantly upregulated upon bacterial infections in respiratory systems [16] , [17] , [18] . In contrast, low expression of CYLD has also been reported in tumours [15] , [19] . Interestingly, under physiological conditions, Cyld-deficient mice exhibited no overt abnormalities and have a normal lifespan [20] . Together, it is evident that maintaining appropriate functional activity and expression of CYLD is critical for tightly controlling overactive inflammation and cell proliferation. Thus, we hypothesized that upregulating expression of CYLD, a key negative regulator of inflammation, for example, by pharmacological inhibition of its own negative regulator, may represent a novel and advantageous anti-inflammatory strategy without causing serious adverse effects often seen with targeting positive regulator of inflammation. Phosphodiesterases (PDEs) have long been thought as attractive and excellent therapeutic targets due to their unique tissue distribution, structural and functional properties, as well as sensitivity to selective inhibitors [21] , [22] . The PDE superfamily comprises 11 subfamilies, named PDE1-PDE11 in mammals [21] , [22] . They act as important positive and negative regulators of cellular response [23] , [24] , [25] , [26] . To date, a number of PDE inhibitors have been already successfully developed as drugs in the clinic, for example, Viagra (targeting PDE5) for erectile dysfunction and Roflumilast (targeting PDE4) for asthma and COPD [21] , [27] . However, the available general PDE4 inhibitors (targeting all of four subfamily members A–D) exhibit serious, sometimes intolerable, adverse effects, for example, emesis, due to its inhibitory effect on PDE4D [21] , [28] , [29] . Moreover, inhibition of PDE4D caused impaired growth [30] . Thus, identifying another PDE4 subfamily member, for example, PDE4B but not PDE4D, as a key regulator and therapeutic target for inflammation may lead to the development of a novel and more tolerable anti-inflammatory agent for treating inflammatory disorders such as OM, a prevalent childhood disease. In the present study, we identified PDE4B as a key negative regulator for CYLD via selective activation of c-jun N-terminal kinase 2 (JNK2), but not JNK1, and inhibition of PDE4B significantly enhanced NTHi-induced CYLD expression and suppressed inflammation. These studies provide insights into the molecular mechanisms underlying the tight regulation of inflammation via inhibition of its negative regulator and may lead to the development of new anti-inflammatory therapeutics via upregulating CYLD expression. PDE4 is a key negative regulator for upregulation of CYLD PDEs have long been thought of as excellent therapeutic targets [21] , [27] . As PDE4 has been shown to have a critical role in mediating immune response, we initially sought to determine whether PDE4 acts as a key negative regulator for CYLD expression. We first evaluated the effects of specific PDE4 inhibitors on the upregulation of CYLD induced by the bacterial pathogen NTHi (clinical strain 12). Interestingly, pharmacologic inhibition of PDE4 using specific PDE4 inhibitor Rolipram markedly enhanced NTHi-induced upregulation of CYLD at both messenger RNA and protein levels in human lung A549, human middle ear HMEEC and human primary bronchial NHBE cells cultured under both conventional and air-liquid interface culture conditions (Fig. 1a–d ). Similarly, Rolipram also enhanced upregulation of CYLD at mRNA and protein levels in the lung and the middle ear mucosa of well-established mouse models of lung inflammation and middle ear inflammation (OM) as assessed by performing real-time quantitative PCR (Q-PCR) and immunofluorescence (IF) staining using CYLD-specific antibody ( Fig. 1e–h ). In addition to Rolipram, Roflumilast, the clinically approved PDE4-specific inhibitor, also significantly enhanced NTHi-induced upregulation of CYLD ( Fig. 1i ). It should be noted that similar results were also observed in the cells treated with three additional commonly used clinical NTHi strains 1479, 2019 and 5657, demonstrating the generalizability of the negative role of PDE4 in regulating CYLD induction by multiple NTHi bacterial strains ( Supplementary Fig. S1 ). Together, our data suggest that PDE4 acts as a key negative regulator of CYLD induction by multiple NTHi strains in human epithelial cells in vitro and in mouse models of both lung and middle ear inflammation. 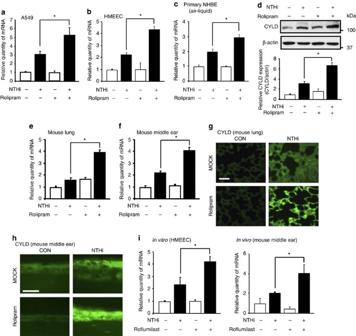Figure 1: PDE4 acts as a key negative regulator for NTHi-induced upregulation of CYLD expression. (a–c) CYLD mRNA expression was measured in (a) human lung A549, (b) human middle ear HMEEC or (c) human primary bronchial NHBE cells pretreated with Rolipram (10 μM) for 1 h and stimulated with NTHi for 5 h. (d) HMEEC cells were pretreated with Rolipram for 1 h, followed by NTHi stimulation, and cell lysates were analysed by immunoblotting with the indicated antibodies (upper panel). CYLD protein expression was quantified from three independent experiments (lower panel). CYLD mRNA expression was measured in (e) lung and (f) middle ear tissues from C57BL/6J mice preinoculated with Rolipram (10 mg/kg) for 2 h and inoculated with NTHi for 9 h. Mouse tissues from (g) lung and (h) middle ear were stained against CYLD after NTHi inoculation, with or without inoculation of Rolipram (magnification × 200 ing; × 400 inh, respectively). Scale bars, 20 μm. (i) CYLD mRNA expression in HMEEC (left panel) or mouse middle ear tissues (right panel) was measured after NTHi treatment, pretreated with or without Roflumilast (1 μM forin vitro, 5 mg/kg forin vivo). Data ina–fandiare mean±s.d. (n=3). *P<0.05. Statistical analysis was performed using Student’st-test. Data are representative of three or more independent experiments. Figure 1: PDE4 acts as a key negative regulator for NTHi-induced upregulation of CYLD expression. ( a – c ) CYLD mRNA expression was measured in ( a ) human lung A549, ( b ) human middle ear HMEEC or ( c ) human primary bronchial NHBE cells pretreated with Rolipram (10 μM) for 1 h and stimulated with NTHi for 5 h. ( d ) HMEEC cells were pretreated with Rolipram for 1 h, followed by NTHi stimulation, and cell lysates were analysed by immunoblotting with the indicated antibodies (upper panel). CYLD protein expression was quantified from three independent experiments (lower panel). CYLD mRNA expression was measured in ( e ) lung and ( f ) middle ear tissues from C57BL/6J mice preinoculated with Rolipram (10 mg/kg) for 2 h and inoculated with NTHi for 9 h. Mouse tissues from ( g ) lung and ( h ) middle ear were stained against CYLD after NTHi inoculation, with or without inoculation of Rolipram (magnification × 200 in g ; × 400 in h , respectively). Scale bars, 20 μm. ( i ) CYLD mRNA expression in HMEEC (left panel) or mouse middle ear tissues (right panel) was measured after NTHi treatment, pretreated with or without Roflumilast (1 μM for in vitro , 5 mg/kg for in vivo ). Data in a – f and i are mean±s.d. ( n =3). * P<0.05 . Statistical analysis was performed using Student’s t- test. Data are representative of three or more independent experiments. Full size image Inhibition of PDE4 suppresses NTHi-induced inflammation We next determined whether PDE4 inhibitor suppresses NTHi-induced inflammation. As expected, the PDE4 inhibitor Rolipram potently inhibited NTHi-induced nuclear factor-κB (NF-κB) activation ( Fig. 2a ) and upregulation of key pro-inflammatory mediators including interleukin (IL)-1β, IL-8 and tumour necrosis factor-α (TNF-α) in A549, HMEEC and primary NHBE cells as assessed by luciferase assay and Q-PCR ( Fig. 2b and Supplementary Fig. S2a ,b). Consistently with its anti-inflammatory effects in vitro , intraperitoneal (i.p.) preadministration of Rolipram also inhibited NTHi-induced upregulation of key pro-inflammatory mediators including MIP-2 (mouse homologue of human IL-8) in the lung and the middle ear of mice ( Fig. 2c ). Moreover, histopathological analysis revealed that Rolipram inhibited NTHi-induced inflammation in both lung and middle ear of mice (Fig. 2e ). In addition, Rolipram also inhibited the middle ear mucosal thickening ( Fig. 2g ) and the typical otoscopic pathological changes of OM including congestion and swelling of the tympanic membrane and mucous effusion accumulation inside the bulla, as assessed by performing otoscopic examination in NTHi-inoculated mice ( Fig. 2h ). Similarly to Rolipram, Roflumilast, also significantly inhibited NTHi-induced inflammation in vitro and in vivo ( Fig. 2i and Supplementary Fig. S2c –e). Collectively, these data demonstrate that inhibition of PDE4 indeed suppressed NTHi-induced inflammatory response in human lung and middle ear epithelial cells in vitro and also in well-established mouse models of lung and middle ear inflammation. 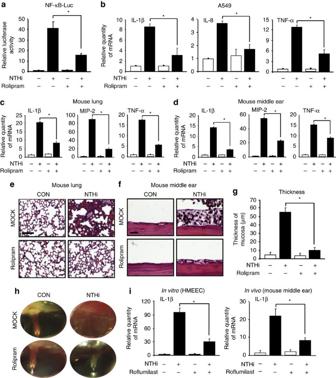Figure 2: Inhibition of PDE4 leads to suppression of NTHi-induced inflammationin vitroandin vivo. (a) A549 cells were pretreated with Rolipram (10 μM) for 1 h, followed by NTHi stimulation, and NF-κB-promoter activity was determined. (b) mRNA expression of pro-inflammatory cytokines was measured in A549 cells pretreated with Rolipram for 1 h and stimulated with NTHi. mRNA expression of pro-inflammatory cytokines was measured in (c) lung and (d) middle ear tissues from C57BL/6J mice preinoculated with Rolipram (10 mg/kg) for 2 h and inoculated with NTHi for 9 h. Haematoxylin and eosin staining of (e) lung and (f) middle ear tissues from C57BL/6J mice preinoculated with Rolipram for 2 h and inoculated with NTHi for 9 h (magnification × 100 ine; × 400 inf, respectively). Scale bars, 100 μm ine; 20 μm inf. (g) Thickness of middle ear mucosa in C57BL/6J mice preinoculated with Rolipram and inoculated with NTHi was measured from 15 middle ear tissue sections per experimental group. (h) Mice were transtympanically inoculated with NTHi with or without Rolipram pretreatment, and tympanic cavity was observed and recorded under the otoscope. (i) IL-1β mRNA expression in HMEEC (left panel) or mouse middle ear tissues (right panel) was measured after NTHi treatment pretreated with or without Roflumilast (1 μM forin vitro, 5 mg kg−1forin vivo). Data ina–d,gandiare mean±s.d. (n=3 ina–d,iand 15 ing). *P<0.05. Statistical analysis was performed using Student’st-test. CON, control. Data are representative of three or more independent experiments. Figure 2: Inhibition of PDE4 leads to suppression of NTHi-induced inflammation in vitro and in vivo. ( a ) A549 cells were pretreated with Rolipram (10 μM) for 1 h, followed by NTHi stimulation, and NF-κB-promoter activity was determined. ( b ) mRNA expression of pro-inflammatory cytokines was measured in A549 cells pretreated with Rolipram for 1 h and stimulated with NTHi. mRNA expression of pro-inflammatory cytokines was measured in ( c ) lung and ( d ) middle ear tissues from C57BL/6J mice preinoculated with Rolipram (10 mg/kg) for 2 h and inoculated with NTHi for 9 h. Haematoxylin and eosin staining of ( e ) lung and ( f ) middle ear tissues from C57BL/6J mice preinoculated with Rolipram for 2 h and inoculated with NTHi for 9 h (magnification × 100 in e ; × 400 in f , respectively). Scale bars, 100 μm in e ; 20 μm in f . ( g ) Thickness of middle ear mucosa in C57BL/6J mice preinoculated with Rolipram and inoculated with NTHi was measured from 15 middle ear tissue sections per experimental group. ( h ) Mice were transtympanically inoculated with NTHi with or without Rolipram pretreatment, and tympanic cavity was observed and recorded under the otoscope. ( i ) IL-1β mRNA expression in HMEEC (left panel) or mouse middle ear tissues (right panel) was measured after NTHi treatment pretreated with or without Roflumilast (1 μM for in vitro , 5 mg kg −1 for in vivo ). Data in a–d , g and i are mean±s.d. ( n =3 in a–d , i and 15 in g ). * P<0.05 . Statistical analysis was performed using Student’s t- test. CON, control. Data are representative of three or more independent experiments. Full size image PDE4 inhibition suppresses inflammation by inducing CYLD Having demonstrated that inhibition of PDE4 enhanced upregulation of CYLD and suppressed NTHi-induced inflammation, it is still unclear whether inhibition of PDE4 suppresses inflammation via upregulating the expression of CYLD, a key negative regulator of inflammation, or via inhibiting key positive regulators of inflammation, for example, IKKβ. We first determined if PDE4 inhibitor still suppresses NTHi-induced inflammation in CYLD-depleted cells. Interestingly, PDE4 inhibitor Rolipram no longer inhibited NTHi-induced upregulation of pro-inflammatory mediators in A549 and HMEEC cells in which CYLD was depleted with CYLD short interfering RNA ( Fig. 3a and Supplementary Fig. S3a ). Similarly, Rolipram also failed to inhibit NTHi-induced mRNA expression of these cytokines in Cyld-deficient mouse embryonic fibroblasts (MEFs) ( Fig. 3b ). Moreover, similar results were also confirmed in mouse models of NTHi-induced inflammation in the lung and middle ear. As shown in Fig. 3c , preadministration (i.p.) of Rolipram no longer inhibited NTHi-induced upregulation of TNF-α and IL-1β in the lung and middle ear of Cyld-deficient mice. As revealed by performing histopathological analysis, Rolipram also failed to suppress NTHi-induced inflammatory response in Cyld-deficient mice as compared with wild-type (WT) mice ( Fig. 3e ). In agreement with these findings, Rolipram also no longer inhibited polymorphonuclear neutrophil infiltration in bronchoalveolar lavage fluids and the middle ear mucosal thickening in Cyld-deficient mice as compared with WT mice ( Fig. 3g and Supplementary Fig. S3b,c ). In addition to Rolipram, Roflumilast also no longer inhibited NTHi-induced upregulation of pro-inflammatory mediators in HMEEC and A549 cells in which CYLD was depleted with CYLD siRNA ( Supplementary Fig. S3d,e ). These data suggest that inhibition of PDE4 indeed suppressed NTHi-induced inflammation in vitro and in vivo via upregulating CYLD expression. 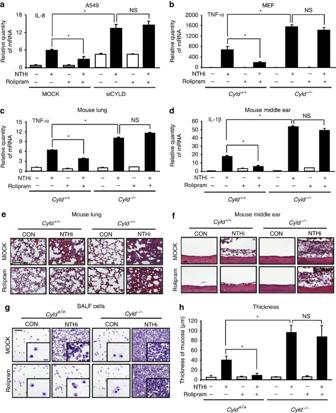Figure 3: Inhibition of PDE4 leads to suppression of NTHi-induced inflammation via upregulation of CYLD expression. (a) A549 cells transfected with siCON or siCYLD were pretreated with Rolipram (10 μM) for 1 h, and IL-8 mRNA expression was measured post NTHi treatment. (b) TNF-α mRNA expression was measured in MEF cells fromCyld+/+andCyld−/−mice pretreated with Rolipram (10 μM) for 1 h and stimulated with NTHi. mRNA expression of pro-inflammatory cytokines was measured in (c) lung and (d) middle ear tissues fromCyld+/+andCyld−/−mice preinoculated with Rolipram (10 mg kg−1, i.p.) for 2 h and inoculated with NTHi. Haematoxylin and eosin staining of (e) lung and (f) middle ear tissues fromCyld+/+andCyld−/−mice preinoculated with Rolipram for 2 h and inoculated with NTHi (magnification × 100 ine; × 400 inf, respectively). Scale bars, 100 μm ine; 20 μm inf. (g) Polymorphonuclear neutrophils (PMNs) were collected from the lung tissues ofCyld+/+andCyld−/−mice preinoculated with Rolipram and inoculated with NTHi by performing bronchoalveolar lavage. PMNs were stained with Diff-Quik staining system after cytocentrifugation (magnification × 100 in large frame; × 400 in inserted frame). Scale bars, 100 μm in large frame; 200 μm in inserted frame. (h) Thickness of middle ear mucosa inCyld+/+andCyld−/−mice preinoculated with Rolipram and inoculated with NTHi was measured from 15 middle ear tissue sections per experimental group. Data ina–dandhare mean±s.d. (n=3 ina–dand 15 inh). *P<0.05. Statistical analysis was performed using Student’st-test. Data are representative of three or more independent experiments. CON, control; NS, nonsignificant. Figure 3: Inhibition of PDE4 leads to suppression of NTHi-induced inflammation via upregulation of CYLD expression. ( a ) A549 cells transfected with siCON or siCYLD were pretreated with Rolipram (10 μM) for 1 h, and IL-8 mRNA expression was measured post NTHi treatment. ( b ) TNF-α mRNA expression was measured in MEF cells from Cyld +/+ and Cyld −/− mice pretreated with Rolipram (10 μM) for 1 h and stimulated with NTHi. mRNA expression of pro-inflammatory cytokines was measured in ( c ) lung and ( d ) middle ear tissues from Cyld +/+ and Cyld −/− mice preinoculated with Rolipram (10 mg kg −1 , i.p.) for 2 h and inoculated with NTHi. Haematoxylin and eosin staining of ( e ) lung and ( f ) middle ear tissues from Cyld +/+ and Cyld −/− mice preinoculated with Rolipram for 2 h and inoculated with NTHi (magnification × 100 in e ; × 400 in f , respectively). Scale bars, 100 μm in e ; 20 μm in f . ( g ) Polymorphonuclear neutrophils (PMNs) were collected from the lung tissues of Cyld +/+ and Cyld −/− mice preinoculated with Rolipram and inoculated with NTHi by performing bronchoalveolar lavage. PMNs were stained with Diff-Quik staining system after cytocentrifugation (magnification × 100 in large frame; × 400 in inserted frame). Scale bars, 100 μm in large frame; 200 μm in inserted frame. ( h ) Thickness of middle ear mucosa in Cyld +/+ and Cyld −/− mice preinoculated with Rolipram and inoculated with NTHi was measured from 15 middle ear tissue sections per experimental group. Data in a – d and h are mean±s.d. ( n =3 in a – d and 15 in h ). * P<0.05 . Statistical analysis was performed using Student’s t- test. Data are representative of three or more independent experiments. CON, control; NS, nonsignificant. Full size image We next determined whether PDE4 inhibitors may also suppress inflammation via directly inhibiting IKKβ, the key positive regulator of NF-κB-dependent inflammation, or p65, the key subunit of NF-κB. As shown in Supplementary Fig. S4a,b , Rolipram did not significantly inhibit activation of NF-κB when induced by overexpressing either a constitutively active form of IKKβ or WT p65. Taken together, our data confirmed our hypothesis that PDE4 acts as a crucial inhibitor for CYLD, a key negative regulator for inflammation. Additionally, we also showed that inhibition of PDE4 using PDE4-specific inhibitors suppresses NTHi-induced inflammation by upregulating expression of CYLD, but not by inhibiting IKKβ or NF-κB p65, the positive regulators of inflammation. PDE4B mediates inflammation by downregulating CYLD We next sought to determine which PDE4 subfamily member is specifically involved in mediating NTHi-induced inflammation by negatively regulating CYLD. PDE4 consists of four subfamily genes, PDE4A to D , encoding Rolipram-sensitive PDEs [27] . PDE4 exerts its cellular functions by catalysing and degrading cyclic AMP (cAMP), one of the important second messengers in regulating numerous pathological processes in response to stimulants, for example, bacterial pathogens [22] . Previous studies indicate that upregulation of PDE4 has an important role in modulating pathological responses [28] , [31] , [32] . Thus, we first determined whether PDE4 is upregulated by NTHi. As shown in Fig. 4a and Supplementary Fig. S5a,b , PDE4B is selectively and markedly upregulated by NTHi at mRNA and protein levels in HMEEC, A549 and primary NHBE cells, in vitro . Similar to the in vitro findings, NTHi-induced upregulation of PDE4B at both mRNA and protein levels was also confirmed in the mouse lung and middle ear in vivo as assessed by performing Q–PCR and IF analysis ( Fig. 4c–f ). Consistent with these results, PDE4B enzymatic activity was also upregulated by NTHi ( Fig. 4g ). Together, these data suggest that PDE4B may have an important role in mediating NTHi-induced inflammation via negative regulation of CYLD. 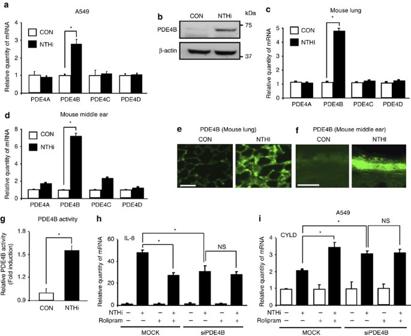Figure 4: PDE4B has a crucial role in mediating NTHi-induced inflammation by negatively regulating CYLD expression. (a) PDE4 mRNA expression was measured in A549 cells stimulated with NTHi for 1.5 h. (b) Cells were treated with NTHi, and cell lysates were analysed by immunoblotting with the indicated antibodies. PDE4 mRNA expression was measured in (c) lung and (d) middle ear tissues from C57BL/6J mice inoculated with NTHi for 4 h. Mouse tissues from (e) lung and (f) middle ear were stained against PDE4B after NTHi inoculation (magnification × 200 ine; × 400 inf, respectively). Scale bars, 20 μm. (g) Lysates from cells treated with NTHi were immunoprecipitated with anti-PDE4B antibody, and analysed by PDE activity assay. (h) Cells transfected with siCON or siPDE4B were pretreated with Rolipram (10 μM) for 1 h, and IL-8 mRNA expression was measured post NTHi treatment. (i) A549 cells transfected with siCON or siPDE4B were pretreated with Rolipram for 1 h, and CYLD mRNA expression was measured post NTHi treatment. Data ina,c,dandg–iare mean±s.d. (n=3). *P<0.05. Statistical analysis was performed using Student’st-test. CON, control. Data are representative of three or more independent experiments. NS, nonsignificant. Figure 4: PDE4B has a crucial role in mediating NTHi-induced inflammation by negatively regulating CYLD expression. ( a ) PDE4 mRNA expression was measured in A549 cells stimulated with NTHi for 1.5 h. ( b ) Cells were treated with NTHi, and cell lysates were analysed by immunoblotting with the indicated antibodies. PDE4 mRNA expression was measured in ( c ) lung and ( d ) middle ear tissues from C57BL/6J mice inoculated with NTHi for 4 h. Mouse tissues from ( e ) lung and ( f ) middle ear were stained against PDE4B after NTHi inoculation (magnification × 200 in e ; × 400 in f , respectively). Scale bars, 20 μm. ( g ) Lysates from cells treated with NTHi were immunoprecipitated with anti-PDE4B antibody, and analysed by PDE activity assay. ( h ) Cells transfected with siCON or siPDE4B were pretreated with Rolipram (10 μM) for 1 h, and IL-8 mRNA expression was measured post NTHi treatment. ( i ) A549 cells transfected with siCON or siPDE4B were pretreated with Rolipram for 1 h, and CYLD mRNA expression was measured post NTHi treatment. Data in a , c , d and g – i are mean±s.d. ( n =3). * P<0.05 . Statistical analysis was performed using Student’s t- test. CON, control. Data are representative of three or more independent experiments. NS, nonsignificant. Full size image We next determined whether PDE4B has an important role in mediating NTHi-induced inflammation by negatively regulating CYLD. We first investigated whether PDE4 inhibitor Rolipram still suppresses NTHi-induced inflammation in PDE4B-depleted cells. As shown in Fig. 4h and Supplementary Fig. S5c–e , Rolipram no longer further inhibited NTHi-induced upregulation of pro-inflammatory mediator IL-1β and IL-8 in HMEEC and A549 cells in which PDE4B was depleted with PDE4B siRNA. Similarly, Rolipram also failed to further enhance NTHi-induced CYLD expression in PDE4B-depleted cells ( Fig. 4i and Supplementary Fig. S5f ). Taken together, our data suggest that PDE4B indeed has a crucial role in mediating NTHi-induced inflammation by negatively regulating CYLD expression. PDE4B downregulates CYLD via activation of JNK2 pathway We next sought to determine how PDE4B mediates NTHi-induced inflammation via negatively regulating CYLD expression. As the mitogen-activated protein kinase (MAPK) JNK has an important role in mediating bacteria-induced host response [33] , [34] , [35] , we initially determined the involvement of JNK in regulating CYLD using specific JNK inhibitor, SP600125. As shown in Fig. 5a , inhibition of JNK using SP600125 markedly enhanced NTHi-induced upregulation of CYLD and suppressed inflammation in HMEEC cells in vitro and in the middle ear of mouse in vivo . Interestingly, PDE4 inhibition using Rolipram no longer enhanced NTHi-induced upregulation of CYLD and suppressed inflammation in HMEEC cells that had been already pretreated with SP600125 ( Fig. 5c ). These results suggest that PDE4B negatively regulates CYLD expression and mediates inflammation via the JNK pathway. 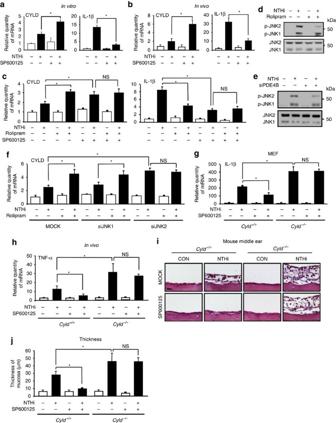Figure 5: PDE4B negatively regulates CYLD expression via specific activation of JNK2 but not JNK1. CYLD and IL-1β mRNA expression was measured in HMEEC (a), mouse middle ear (b) pretreated with SP600125 (5 μM for 1 hin vitro, 5 mg kg−1for 2 hin vivo) and stimulated with NTHi. (c) CYLD, IL-1β mRNA expression in cells was measured after NTHi stimulation pretreated with Rolipram (10 μM) and SP600125 (5 μM). (d) Cells were pretreated with Rolipram, followed by NTHi stimulation, and cell lysates were analysed by immunoblotting with the indicated antibodies. (e) Cells were transfected with siCON or siPDE4B, followed by NTHi stimulation, and cell lysates were analysed by immunoblotting with the indicated antibodies. (f) Cells transfected with siCON, siJNK1 or siJNK2 were pretreated with Rolipram (10 μM), and CYLD mRNA expression was measured post NTHi treatment. (g) IL-1β mRNA expression was measured in MEF cells fromCyld+/+,Cyld−/−mice after NTHi stimulation pretreated with SP600125 (5 μM). (h) TNF-α mRNA expression was measured in middle ear tissues fromCyld+/+,Cyld−/−mice preinoculated with SP600125 (5 mg kg−1) and inoculated with NTHi. (i) Haematoxylin and eosin staining of middle ear tissues fromCyld+/+,Cyld−/−mice preinoculated with SP600125 and inoculated with NTHi (magnification × 400). Scale bars, 20 μm. (j) Thickness of middle ear mucosa inCyld+/+,Cyld−/−mice preinoculated with SP600125 and inoculated with NTHi was measured from 15 middle ear tissue sections per experimental group. Data ina–c,f–handjare mean±s.d. (n=3 ina–c,f–hand 15 inj). *P<0.05. Statistical analysis was performed using Student’st-test. Data are representative of three or more independent experiments. CON, control; NS, nonsignificant. Figure 5: PDE4B negatively regulates CYLD expression via specific activation of JNK2 but not JNK1. CYLD and IL-1β mRNA expression was measured in HMEEC ( a ), mouse middle ear ( b ) pretreated with SP600125 (5 μM for 1 h in vitro , 5 mg kg −1 for 2 h in vivo ) and stimulated with NTHi. ( c ) CYLD, IL-1β mRNA expression in cells was measured after NTHi stimulation pretreated with Rolipram (10 μM) and SP600125 (5 μM). ( d ) Cells were pretreated with Rolipram, followed by NTHi stimulation, and cell lysates were analysed by immunoblotting with the indicated antibodies. ( e ) Cells were transfected with siCON or siPDE4B, followed by NTHi stimulation, and cell lysates were analysed by immunoblotting with the indicated antibodies. ( f ) Cells transfected with siCON, siJNK1 or siJNK2 were pretreated with Rolipram (10 μM), and CYLD mRNA expression was measured post NTHi treatment. ( g ) IL-1β mRNA expression was measured in MEF cells from Cyld +/+ , Cyld −/− mice after NTHi stimulation pretreated with SP600125 (5 μM). ( h ) TNF-α mRNA expression was measured in middle ear tissues from Cyld +/+ , Cyld −/− mice preinoculated with SP600125 (5 mg kg −1 ) and inoculated with NTHi. ( i ) Haematoxylin and eosin staining of middle ear tissues from Cyld +/+ , Cyld −/− mice preinoculated with SP600125 and inoculated with NTHi (magnification × 400). Scale bars, 20 μm. ( j ) Thickness of middle ear mucosa in Cyld +/+ , Cyld −/− mice preinoculated with SP600125 and inoculated with NTHi was measured from 15 middle ear tissue sections per experimental group. Data in a – c , f – h and j are mean±s.d. ( n =3 in a – c , f – h and 15 in j ). * P<0.05 . Statistical analysis was performed using Student’s t- test. Data are representative of three or more independent experiments. CON, control; NS, nonsignificant. Full size image As JNK1 and 2 represent the two major isoforms expressed in the middle ear and lung epithelial cells, we next determined which isoform is involved. Interestingly, PDE4 inhibitor selectively suppressed NTHi-induced activation of JNK2, but not JNK1 ( Fig. 5d ). We further determined whether PDE4B mediates the selective activation of JNK2 induced by NTHi using siRNA PDE4B. As shown in Fig. 5e , PDE4B knockdown selectively inhibited activation of JNK2 but not JNK1, thereby confirming that PDE4B negatively regulates NTHi-induced CYLD expression and mediates inflammation via specific activation of JNK2 but not JNK1. Having established that JNK2 acts downstream of PDE4B in negatively regulating CYLD expression and mediating NTHi-induced inflammation, we sought to determine whether JNK2 indeed acts upstream of CYLD to mediate PDE4B-dependent NTHi-induced inflammation. As shown in Fig. 5f and Supplementary Fig. S6 , inhibition of PDE4 using Rolipram still enhanced NTHi-induced upregulation of CYLD in JNK1-depleted cells but not in JNK2-depleted cells, confirming the selective requirement of JNK2 in mediating PDE4B-depenent negative regulation of CYLD expression. We next investigated whether JNK2 pathway indeed regulates NTHi-induced inflammation in a CYLD-dependent manner using Cyld-deficient cells and mice. As expected, NTHi-induced inflammation was significantly enhanced in Cyld-deficient cells and the JNK inhibitor no longer inhibited NTHi-induced inflammation in Cyld-deficient cells as compared with WT cells ( Fig. 5g ). Consistent with these in vitro findings, i.p. preadministration of SP600125 inhibited NTHi-induced upregulation of the key pro-inflammatory mediators in the middle ear of WT mice but not in Cyld-deficient mice ( Fig. 5h ). Similarly, histopathological analysis revealed that SP600125 also failed to inhibit NTHi-induced middle ear inflammation including mucosal thickening in Cyld-deficient mice (Fig. 5i ). Taken together, it is evident that PDE4B negatively regulates CYLD expression and mediates NTHi-induced inflammation via specific activation of JNK2 but not JNK1 pathway. PDE4B activates JNK2 by inhibiting cAMP-PKA pathway PDE4 exerts its effects by catalysing and degrading cAMP and thereby tightly controlling its intracellular concentrations [21] . Inhibition of PDE4 activity leads to an increase in intracellular concentration of cAMP. Thus, we sought to determine whether increased cAMP does have an important role in inhibiting JNK2 activation, which in turn enhances CYLD expression and suppresses inflammation. We first evaluated the effect of 8-bromo-cAMP (8-Br-cAMP), a cell-permeable cAMP analogue which is more resistant to PDE4 than cAMP, on NTHi-induced JNK activation. Similarly to the effect of PDE4 inhibition, 8-Br-cAMP selectively inhibited NTHi-induced activation of JNK2 but not JNK1 in HMEEC cells ( Fig. 6a ). We further confirmed the involvement of cAMP in NTHi-induced JNK2 activation by using Forskolin, a cell-permeable diterpenoid, which has been commonly used to increase levels of intracellular cAMP. As shown in Fig. 6b , Forskolin inhibited NTHi-induced activation of JNK2 but not JNK1. As protein kinase A (PKA) represents the major downstream signalling effector of cAMP, and PKA was known to be involved in regulating inflammation, we next determined whether cAMP-dependent PKA pathway is critically involved in NTHi-induced JNK2 activation by using PKA inhibitor (PKI). As shown in Fig. 6c , PKI enhanced NTHi-induced activation of JNK2 but not JNK1. Together, these data suggest that cAMP-dependent PKA pathway has an important role in mediating NTHi-induced JNK2 activation. We next determined whether cAMP-dependent PKA pathway also has a critical role in mediating NTHi-induced CYLD expression and inflammation. As shown in Fig. 6d–f , 8-Br-cAMP and Forskolin enhanced, whereas PKI inhibited, NTHi-induced upregulation of CYLD expression in HMEEC cells. Consistent with these results, 8-Br-cAMP and Forskolin inhibited, whereas PKI enhanced, NTHi-induced upregulation of IL-1β in HMEEC cells ( Fig. 6g–i ). Collectively, our data suggest that PDE4B selectively mediates NTHi-induced JNK2 activation via inhibition of cAMP-PKA-dependent pathway, which in turn leads to suppression of CYLD and subsequent induction of inflammation ( Fig. 6j ). Interestingly, the basal expression level of CYLD is elevated by Forskolin and 8-Br-cAMP but not Rolipram. This discrepancy is likely due to the difference in the elevated subcellular pools of cAMP. Forskolin is known to activate a number of adenylyl cyclases and elevates a wider range of subcellular pools of cAMP. 8-Br-cAMP is a non-hydrolysable cAMP analogue resistant to PDEs. In contrast, Rolipram is a selective inhibitor for PDE4, particularly PDE4B, which hydrolyses cAMP in more restricted subcellular compartments. These results suggest the involvement of additional mechanism to induce CYLD. In addition, how CYLD mRNA expression is increased upon treatment involving cAMP, through inhibition of JNK2 or not, remains unknown. Future studies are warranted to further elucidate the underlying mechanisms by determining the effects of specific depletion of JNK1 or 2 or both in cAMP-mediated CYLD expression. 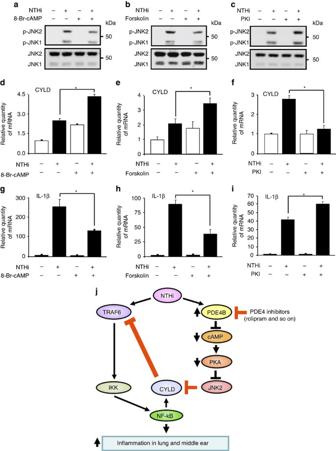Figure 6: PDE4B activates JNK2 leading to suppression of CYLD and subsequent induction of inflammation. (a–c) Cells were pretreated with (a) 100 μM 8-Br-cAMP, (b) 10 μM Forskolin or (c) 1 μM PKI for 1 h, followed by NTHi stimulation, and cell lysates were analysed by immunoblotting with the indicated antibodies. (d–f) Cells were pretreated with (d) 8-Br-cAMP, (e) Forskolin or (f) PKI for 1 h, followed by NTHi stimulation, and CYLD mRNA expression was measured. (g–i) Cells were pretreated with (g) 8-Br-cAMP, (h) Forskolin or (i) PKI for 1 h, followed by NTHi stimulation, and IL-1β mRNA expression was measured. (j) A schematic model illustrating that PDE4B selectively mediates NTHi-induced JNK2 activation via inhibition of cAMP-PKA-dependent pathway, which in turn leads to suppression of CYLD and subsequent induction of inflammation. Data ind–iare mean±s.d. (n=3). *P<0.05. Statistical analysis was performed using Student’st-test. Data are representative of three or more independent experiments. Figure 6: PDE4B activates JNK2 leading to suppression of CYLD and subsequent induction of inflammation. ( a – c ) Cells were pretreated with ( a ) 100 μM 8-Br-cAMP, ( b ) 10 μM Forskolin or ( c ) 1 μM PKI for 1 h, followed by NTHi stimulation, and cell lysates were analysed by immunoblotting with the indicated antibodies. ( d – f ) Cells were pretreated with ( d ) 8-Br-cAMP, ( e ) Forskolin or ( f ) PKI for 1 h, followed by NTHi stimulation, and CYLD mRNA expression was measured. ( g – i ) Cells were pretreated with ( g ) 8-Br-cAMP, ( h ) Forskolin or ( i ) PKI for 1 h, followed by NTHi stimulation, and IL-1β mRNA expression was measured. ( j ) A schematic model illustrating that PDE4B selectively mediates NTHi-induced JNK2 activation via inhibition of cAMP-PKA-dependent pathway, which in turn leads to suppression of CYLD and subsequent induction of inflammation. Data in d – i are mean±s.d. ( n =3). * P<0.05 . Statistical analysis was performed using Student’s t- test. Data are representative of three or more independent experiments. Full size image Ototopical PDE4 inhibitor suppresses inflammation We have shown that upregulating expression of CYLD, a key negative regulator of inflammation, via inhibition of its own negative regulator, PDE4B, leads to the suppression of NTHi-induced inflammation. We have already demonstrated that specific PDE4 inhibitors, Rolipram and Roflumilast, when preadministered systemically, upregulated CYLD and suppressed subsequent inflammation in the mouse models of middle ear inflammation (OM) and lung inflammation ( Figs 1 and 2 ). These encouraging data thus prompted us to directly test whether post-inoculation administration of Rolipram has any therapeutic effect on treating middle ear inflammation under clinically relevant condition. Ototopical administration works effectively when the eardrum is perforated either pathologically or surgically by tympanostomy tube insertion [36] , [37] , [38] . Thus, we next evaluated whether ototopical administration of Rolipram upregulates CYLD and suppresses inflammation in the middle ear of mice post NTHi infection. Interestingly, both ototopical pre- and post-inoculation administration of Rolipram upregulated CYLD expression ( Fig. 7a ) and suppressed inflammation in a mouse OM model in vivo ( Fig. 7b–e ). Taken together, these data demonstrate that upregulating CYLD expression via pharmacologic inhibition of PDE4 does exhibit significant therapeutic effects in treating inflammatory diseases such as middle ear inflammation (OM). 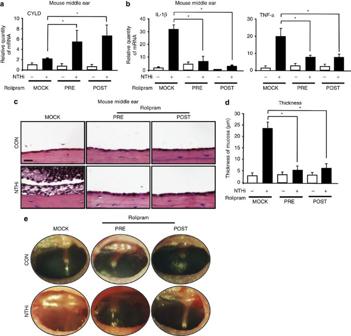Figure 7: Administration of specific PDE4 inhibitors upregulates CYLD and suppresses inflammation in a mouse otitis media model. mRNA expression of (a) CYLD and (b) pro-inflammatory cytokines was measured in middle ear tissues from C57BL/6J mice ototopically pre- or post-inoculated with Rolipram (50 μg per ear) 3 h before (pretreatment) or 3 h after (post treatment) NTHi inoculation, and inoculated with NTHi for 9 h. (c) Haematoxylin and eosin staining of middle ear tissues from C57BL/6J mice ototopically pre- or post-inoculated with Rolipram (50 μg per ear) 3 h before (pretreatment) or 3 h after (post treatment) NTHi inoculation, and inoculated with NTHi for 9 h (magnification × 400). Scale bar, 20 μm. (d) Thickness of middle ear mucosa in C57BL/6J mice ototopically pre- or post-inoculated with Rolipram and inoculated with NTHi was measured from 15 middle ear tissue sections per experimental group. (e) Mice were transtympanically inoculated with NTHi with or without Rolipram ototopically pre- or post-treatment, and tympanic cavity was observed and recorded under the otoscope. Data ina,banddare mean±s.d. (n=3 inaandb, and 15 ind). *P<0.05. Statistical analysis was performed using Student’st-test. Data are representative of three or more independent experiments. CON, control; POST, post-inoculation; PRE, preinoculation. Figure 7: Administration of specific PDE4 inhibitors upregulates CYLD and suppresses inflammation in a mouse otitis media model. mRNA expression of ( a ) CYLD and ( b ) pro-inflammatory cytokines was measured in middle ear tissues from C57BL/6J mice ototopically pre- or post-inoculated with Rolipram (50 μg per ear) 3 h before (pretreatment) or 3 h after (post treatment) NTHi inoculation, and inoculated with NTHi for 9 h. ( c ) Haematoxylin and eosin staining of middle ear tissues from C57BL/6J mice ototopically pre- or post-inoculated with Rolipram (50 μg per ear) 3 h before (pretreatment) or 3 h after (post treatment) NTHi inoculation, and inoculated with NTHi for 9 h (magnification × 400). Scale bar, 20 μm. ( d ) Thickness of middle ear mucosa in C57BL/6J mice ototopically pre- or post-inoculated with Rolipram and inoculated with NTHi was measured from 15 middle ear tissue sections per experimental group. ( e ) Mice were transtympanically inoculated with NTHi with or without Rolipram ototopically pre- or post-treatment, and tympanic cavity was observed and recorded under the otoscope. Data in a , b and d are mean±s.d. ( n =3 in a and b , and 15 in d ). * P<0.05 . Statistical analysis was performed using Student’s t- test. Data are representative of three or more independent experiments. CON, control; POST, post-inoculation; PRE, preinoculation. Full size image In the present study, we showed that inhibition of PDE4B markedly enhanced upregulation of CYLD expression by the bacterial pathogen NTHi, thereby suggesting that PDE4B acts as a negative regulator for CYLD. Interestingly, inhibition of PDE4B no longer suppressed NTHi-induced inflammation in Cyld-deficient cells and mice. Moreover, PDE4B negatively regulates CYLD via selective activation of JNK2 but not JNK1. Importantly, ototopical post-inoculation administration of specific inhibitors for PDE4 suppressed NTHi-induced inflammation in a well-established mouse model of middle ear inflammation, thus demonstrating their therapeutic potential. Our studies offer novel insights into how inflammation is tightly regulated via inhibition of the expression level of CYLD, a key negative regulator for inflammation and may also lead to the development of new anti-inflammatory therapeutics by increasing the expression level of CYLD. Of particular translational and therapeutic significance is that upregulating the expression level of CYLD, a key negative regulator of inflammation, via inhibition of its own negative regulator, PDE4B, resulted in the suppression of bacteria-induced inflammation in well-established mouse models of lung and middle ear inflammation. In reviewing the past therapeutic strategies in developing anti-inflammatory agents, significant efforts have been focused on suppressing inflammation by directly targeting the positive signalling pathways [7] . For instance, suppressing IKKβ using small molecule inhibitors has been one of the focuses [39] . Although these agents exhibited certain efficacy, they, however, often resulted in significant adverse effects, for example, suppression of immune response, impairment of host defence and induction of apoptosis, which prevented their further clinical use in particular for long-term treatment [8] , [9] . Thus, there is an urgent need for developing novel therapeutic strategies without causing serious side effects, by targeting the negative instead of positive regulators of inflammation. Among all known negative regulators of inflammation, deubiquitinase CYLD has been shown to act as a key inducible negative feedback regulator for tightly controlling bacteria-induced inflammation, and thus preventing an overactive response in inflammatory diseases such as COPD and OM [10] , [11] . CYLD suppresses NF-κB-dependent inflammation by removing K63-linked polyubiquitin chains from TRAF2, TRAF6, NEMO, TAK1, Bcl3 and RIP1 (ref. 13 ). In addition to regulating NF-κB-dependent inflammation, CYLD has also been implicated in a number of other cellular responses by targeting MAPK, JNK and p38, Akt, TCR signalling, cell cycle, calcium signalling and antiviral signalling pathways [12] , [13] . Mutations of CYLD have been reported to lead to the development of tumours such as CYLD [14] , [15] . In addition to mutations, dysregulated expression of CYLD has also been reported under various pathological conditions. We previously found that the expression of CYLD is relatively low under physiological conditions but is markedly upregulated by inflammatory insults such as NTHi [16] , [17] , [18] . In contrast, low expression of CYLD has also been reported in tumours [15] , [19] . Interestingly, Cyld knockout mice exhibited no overt abnormalities and a normal lifespan [20] . Thus, it is plausible that increasing the expression level of CYLD by pharmacological inhibition of its own negative regulator may represent a novel and advantageous strategy for treating an overactive response in chronic inflammatory diseases without causing serious adverse effects often seen with targeting a positive regulator of inflammation. Indeed, in our present study, we provided direct in vitro and in vivo evidence for suppressing inflammation by upregulating the expression level of CYLD via specific inhibition of its own negative regulator PDE4B. It should be noted that inhibition of PDE4B via post-inoculation administration of PDE4 inhibitor also exhibited significant therapeutic effects on suppressing bacteria-induced inflammation in a well-established mouse model of middle ear inflammation. Our studies may provide novel therapeutic strategies for suppressing inflammation via directly upregulating its the negative regulators instead of inhibiting the positive regulators, thereby avoiding the serious side effects often seen when directly inhibiting positive pathway such as IKKβ. In addition to treating inflammatory diseases, upregulating the expression level of CYLD may also lead to promising therapeutic strategies for tumours and fibrosis as the low expression of CYLD has been reported to have an important role in the development of tumours and lung fibrosis in patients. Another major interesting finding in our studies is the identification of PDE4B as a critical negative regulator for upregulation of CYLD expression induced by bacteria. PDEs act as important regulators that both positively and negatively regulate cellular response via controlling the intracellular levels of second messengers cAMP and cGMP [23] , [24] , [25] , [26] . PDEs have long been thought as attractive and excellent therapeutic targets because of their unique tissue distribution, structural and functional properties, as well as sensitivity to selective inhibitors [21] , [22] . Indeed, a number of PDE inhibitors have been already successfully developed as drugs in clinic, for example, Viagra (targeting PDE5) for erectile dysfunction and Roflumilast (targeting PDE4) for asthma and COPD [21] , [27] . However, the available general PDE4 inhibitors exhibited serious, sometimes intolerable, adverse effects due to its inhibitory effect on PDE4D [29] . The major side effects caused by inhibition of PDE4D include severe nausea, emesis and diarrhoea [21] , [28] , [29] . Moreover, inhibition of PDE4D also caused impaired growth [30] . Unfortunately, Roflumilast, the currently available drug, inhibits all of the four isotypes, A–D. Interestingly, our present study provides clear evidence that PDE4B acts as a key negative regulator for CYLD expression in vitro and in vivo . Inhibition of PDE4B markedly increased the expression of CYLD and subsequently suppressed bacteria-induced inflammation in well-established models of both lung and middle ear inflammation. Our studies may lead to the development of novel and more tolerable anti-inflammatory agent by selectively and specifically targeting PDE4B but not PDE4D for treating inflammatory disorders such as OM, which is extremely critical for children. In addition, our encouraging findings also showed that ototopical post-inoculation administration of PDE4 inhibitors significantly suppressed bacteria-induced inflammation. Thus, topical application of currently available drug Roflumilast may allow immediate and broad clinical application to treat inflammatory diseases to minimize the side effects caused due to systemic administration. Of additional biological significance is our finding showing that PDE4B acts as a negative regulator for CYLD expression via selective activation of JNK2 but not JNK1. JNK family of MAPK has been shown to have a critical role in regulating a variety of both physiological and pathological responses [33] , [34] , [35] , [40] . JNK1 and JNK2 represent the major subfamily members of JNK. A number of studies indicate the functional differences and redundancy of JNK1 and JNK2 [40] , [41] , [42] , [43] , [44] . However, how JNK1 and 2 are selectively activated still remains largely unknown. In the present study, we provide direct evidence for the first time that PDE4B specifically and selectively mediates NTHi-induced activation of JNK2 but not JNK1 via a cAMP-PKA-dependent manner, which in turn leads to the negative regulation of CYLD expression. Thus, these studies may bring new insights into the upstream signalling mechanisms underlying specific and selective activation of JNK in inflammatory and infectious diseases. Reagents and antibodies Rolipram, 8-Br-cAMP, forskolin and cyclic nucleotide PDE assay kit were purchased from Enzo Life Sciences. PKI was purchased from EMD Millipore. SP600125 was purchased from A.G. Scientific. Roflumilast was purchased from Santa Cruz Biotechnology. Antibodies against phospho-stress-activated protein kinase/JNK (Thr-183/Tyr-185) and stress-activated protein kinase/JNK were purchased from Cell Signaling Technology. Antibody against CYLD was purchased from IMGENEX Corp. Antibodies against PDE4B and β-actin were purchased from Santa Cruz Biotechnology. Bacterial strains and culture condition Clinical isolates of NTHi strain 12 and three other NTHi strains were used in this study [45] , [46] . Bacteria were grown on chocolate agar plate at 37 °C in an atmosphere of 5% CO 2 overnight and inoculated in brain heart infusion broth supplemented with 3.5 μg ml −1 NAD and hemin. After overnight incubation, bacteria were subcultured into 5 ml of fresh BHI and the log phase NTHi, monitored by measurement of optical density value, was washed and suspended in phosphate-buffered saline (PBS) for in vitro cell experiments and in isotonic saline for in vivo animal experiments. Cell culture All media described below were supplemented with 10% fetal bovine serum (Sigma-Aldrich) and Pen/Strep (100 units per ml penicillin and 0.1 mg per ml streptomycin; Gibco). Human middle ear epithelial HMEEC cells were maintained in DMEM (Cellgro) supplemented with BEGM SingleQuots (Lonza). Human airway epithelial A549 cells were maintained in F-12K medium (Gibco) as described previously [45] , [46] . Human primary bronchial epithelial NHBE (Lonza) cells were maintained in bronchial epithelial growth media (BEGM) supplemented with BEGM SingleQuots [12] . Air–liquid culture of human primary NHBE cells was conducted as described previously [47] . Wild-type (WT) and Cyld −/− MEF cells were obtained from E13 embryos and maintained in DMEM. WT and Cyld −/− MEFs and mice were obtained as described previously [12] , [20] . All cells were cultured in a humidified atmosphere of 5% CO 2 at 37 °C. Real-time quantitative RT–PCR analysis Total RNA was isolated with TRIzol reagent (Invitrogen) by following the manufacturer’s instruction. For the reverse transcription reaction, TaqMan reverse transcription reagents (Applied Biosystems) were used as described [18] , [47] . PCR amplifications were performed by using SYBR Green Universal Master Mix (Applied Biosystems). In brief, reactions were performed in triplicate containing 2 × universal master mix, 1 μl of template cDNA, 500 nM primers in a final volume of 12.5 μl, and they were analysed in a 96-well optical reaction plate (Applied Biosystems). Reactions were amplified and quantified by using an ABI 7500 sequence detector and the manufacturer’s corresponding software (7000v1.3.1; Applied Biosystems). The relative quantities of mRNAs were obtained by using the comparative Ct method and were normalized using human cyclophilin or mouse glyceraldehydes-3-phosphate dehydrogenase as an endogenous control. The primers for human IL-1β, IL-8, TNF-α, CYLD, PDE4A, PDE4B, JNK1, JNK2 and cyclophilin, as well as mouse IL-1β, MIP-2, TNF-α, CYLD, PDE4A, PDE4B and glyceraldehydes-3-phosphate dehydrogenase were described previously [16] , [32] , [35] , [48] . Human PDE4C: 5′-GACTTACCCCTCGACAACCA-3′ and 5′-GAAAGTCTGCCTGCCAAGAG-3′; human PDE4D: 5′-TGCCATCTGTTGATCAGGAA-3′ and 5′-CCCAGTTGTGTTTCCGAGTT-3′; mouse PDE4C: 5′-CATGCAGTCGGACTCTGTGT-3′ and 5′-GGACTGGTGAAGGCAACATT-3′; mouse PDE4D: 5′-CTCTGTGCACCCAAGACTCA-3′ and 5′-CAAGTTTCAGGCTGGCTTTC-3′. Plasmids, transfections and luciferase assay The expression plasmids p65 WT, a constitutively active form of IKKβ (IKKβ-CA), and the luciferase reporter construct of NF-κB were previously described [49] , [50] . Empty vector was used as a control and was also added where necessary to ensure an equivalent amount of input DNA. All transient transfections were carried out in triplicate using TransIT-LT1 reagent (Mirus) following the manufacturer’s instruction. For experiments with inhibitors, the transfected cells were pretreated with or without chemical inhibitors for 1 h followed by 5-h incubation with NTHi lysates. Luciferase activity was normalized with respect to β-galactosidase activity. Data from all experiments are presented as the relative luciferase activity (mean±s.d.) from at least three independent sets of experiments, each with triplicate measurements. RNA-mediated interference RNA-mediated interference for downregulating CYLD expression was carried out using pSUPER-CYLD as described previously [16] , [18] and the sequence for the siCYLD is 5′-GATCCCCGAGCTACTGAGGACAGAAATTCAAGAGATTTCTGTCCTCAGTAGCTCTTTTTGGAAA-3′. Human siRNAs for PDE4B, JNK1 and JNK2 were purchased from Dharmacon, and knockdown of PDE4B, JNK1 and JNK2, using siPDE4B, siJNK1 and siJNK2, was performed using Lipofectamine 2000 (Invitrogen) following the manufacturer’s instruction. ON-TARGETplus SMARTpool of siRNAs targeting human PDE4B, human JNK1 and human JNK2 consists of four siRNAs and sequences for the siRNAs are as follows: Human siPDE4B (5′-AGUUACAAGUUCAGGCGUU-3′, 5′-GCUCAGGACAUUCUCGAUA-3′, 5′-AGACAAUGGUAGAAACGAA-3′, 5′-GCAUUCAGGUCCUUCGCAA-3′); human siJNK1 (5′-GAUGACGCCUUAUGUAGUG-3′, 5′-GAAUAGUAUGCGCAGCUUA-3′, 5′-GGCAUGGGCUACAAGGAAA-3′, 5′-GCCCAGUAAUAUAGUAGUA-3′); human siJNK2 (5′-GAUUGUUUGUGCUGCAUUU-3′, 5′-GGCUGUCGAUGAUAGGUUA-3′, 5′-AGCCAACUGUGAGGAAUUA-3′, 5′-UCGUGAACUUGUCCUCUUA-3′). Western blot analysis Western blot analysis was performed as described previously and following the manufacturer’s instruction [18] . Western blots were performed using whole-cell extracts, separated on 6 or 8% SDS–polyacrylamide gel electrophoresis gels, and transferred to polyvinylidene difluoride membranes. The membrane was blocked with a solution of Tris-buffered saline (TBS) containing 0.1% Tween 20 (TBS-T) and 5% non-fat dry milk. The membrane was then incubated in a 1:2,000 dilution of a primary antibody in 5% BSA-TBS-T. After three washes in TBS-T, the membrane was incubated with 1:5,000 dilution of the corresponding secondary antibody in 5% non-fat dry milk-TBS-T. Respective proteins were visualized by using Amersham ECL Prime Regent (GE Healthcare Biosciences). Immunoprecipitation and PDE assay To conduct the selective immunoprecipitation of PDE4B, cell lysates were incubated with 1 μg of primary antibodies overnight at 4 °C, followed by 2-h incubation with protein A/G-agarose beads (Santa Cruz Biotechnology). Immunoprecipitates were washed three times with PBS and one time with PDE assay buffer (10 mM Tris–HCl, pH 7.4), and then used for PDE assay. PDE activity was measured by using cyclic nucleotide PDE assay kit (Enzo Life Sciences) following the instructions. PDE activity of PDE4B immunoprecipitates was blocked in the presence of 10 μM Rolipram. Mice and animal experiments Cyld −/− mice have been described previously [12] , [20] , and age-matched background C57BL/6J mice were used as WT controls. For NTHi-induced inflammation in WT and Cyld −/− mice, anaesthetized mice were transtympanically or intratracheally inoculated with NTHi at a concentration of 1 × 10 7 or 5 × 10 7 c.f.u. per mouse, respectively, and saline was inoculated as control. The inoculated mice were then killed 9 h after NTHi inoculation. Eardrums of mice were inspected for signs of middle ear inflammation and photographed for recording pathological changes of eardrum under the otoscope. Dissected temporal bones and lungs were then subjected to total RNA extraction and histological analysis. For polymorphonuclear neutrophil analysis, bronchoalveolar lavage was performed by cannulating the trachea with sterilized PBS in WT and Cyld −/− mice [17] . For inhibition study, mice were pretreated with chemical inhibitors i.p. 2 h before NTHi inoculation. For the ototopical pretreatment experiments, mice were pretreated with Rolipram through tympanic membrane 3 h before NTHi inoculation, and inoculated with NTHi for 9 h. For the ototopical post-treatment experiments, mice were inoculated with NTHi first, and ototopically post-treated with Rolipram through tympanic membrane 3 h after NTHi inoculation. The inoculated mice were killed 9 h after NTHi inoculation. All animal experiments were approved by the Institutional Animal Care and Use Committee at Georgia State University. Histology and IF assay For histological analysis, formalin-fixed paraffin-embedded lung and middle ear tissues were sectioned (4 μm), and then stained with haematoxylin and eosin to visualize inflammatory responses and pathological changes in the middle ear or lung. IF detection of CYLD and PDE4B proteins were performed using rabbit anti-CYLD, rabbit anti-PDE4B and FITC-conjugated goat anti-rabbit IgG (Santa Cruz Biotechnology) in the paraffin section of mouse middle ear or lung tissue. Stained sections were then imaged, and images were recorded under light and fluorescence microscopy systems (AxioVert 40 CFL, AxioCam MRC and AxioVision LE Image system, Carl Zeiss). Measurement of mucosal thickness in the middle ear Mucosal thickness in the middle ear cavity was measured from 15 sections per each experimental group using AxioVision LE Image system software (Carl Zeiss) to measure and quantify the degree of inflammation such as mucosal hyperplasia and inflammatory cell infiltration. The average of mucosal thickness from 15 sections was presented in a bar graph as the mean±s.d. along with representative tissue sections. Statistical analysis All experiments were repeated at least three times with consistent results. Data are shown as mean±s.d. Statistical analysis was assessed by two-tailed unpaired student’s t- test. P<0.05 was considered statistically significant. How to cite this article: Komatsu, K. et al . Inhibition of PDE4B suppresses inflammation by increasing expression of the deubiquitinase CYLD. Nat. Commun. 4:1684 doi: 10.1038/ncomms2674 (2012).